Structure and mechanism of a canonical poly(ADP-ribose) glycohydrolase Poly(ADP-ribosyl)ation is a reversible post-translational protein modification involved in the regulation of a number of cellular processes including DNA repair, chromatin structure, mitosis, transcription, checkpoint activation, apoptosis and asexual development. The reversion of poly(ADP-ribosyl)ation is catalysed by poly(ADP-ribose) (PAR) glycohydrolase (PARG), which specifically targets the unique PAR (1′′-2′) ribose–ribose bonds. Here we report the structure and mechanism of the first canonical PARG from the protozoan Tetrahymena thermophila . In addition, we reveal the structure of T. thermophila PARG in a complex with a novel rhodanine-containing mammalian PARG inhibitor RBPI-3. Our data demonstrate that the protozoan PARG represents a good model for human PARG and is therefore likely to prove useful in guiding structure-based discovery of new classes of PARG inhibitors. PAR is synthesized by the PARP family of enzymes in a reaction that utilizes NAD as a substrate. In contrast to the abundance of structural and functional data describing PAR synthesis [1] , [2] , [3] , [4] , our present understanding of the PAR-degradation pathway is comparatively poor [5] , [6] . Canonical PARG is a highly conserved protein found in organisms ranging from protozoa to humans [7] . The disruption of the PARG gene in mouse and Drosophila melanogaster leads to early embryonic lethality [8] , [9] . A highly diverged PARG (bacterial-type) is present in filamentous fungi and a number of bacterial species [10] . The recently solved structure of a bacterial PARG revealed that the catalytic centre is essentially a macrodomain with a loop region inserted that contains the PARG signature sequence (GGG-X 6−8 -QEE) [5] , [10] . Macrodomains are evolutionarily conserved ADP-ribose-binding modules that often mediate PAR signalling [11] , [12] , [13] . The bacterial PARG structures combined with biochemical studies established a role for the PARG signature residues in substrate binding and catalysis [10] . Despite this progress, structural information on the canonical PARGs is still lacking. Recent studies identified a minimal region in human PARG required for catalytic activity in vitro , which extends beyond the macrodomain alone [14] . This amino-terminal extension contains a short motif called the Regulatory Segment/MTS (RS/MTS) that was suggested to be essential for PARG activity [14] . Additionally, a conserved tyrosine only present in canonical-type PARGs (Y795 in human PARG) was suggested to be involved in PAR binding [15] . To investigate the mechanism and structure of canonical-type PARGs, we screened for a crystallizable homologue of the human PARG catalytic core, and identified a PARG from the ciliated protozoan Tetrahymena thermophila (TTPARG). Our structures of TTPARG in complex with ADP-ribose and the mammalian PARG inhibitor RBPI-3 combined with solution studies reveal details of the substrate recognition and the reaction mechanism of canonical PARGs. The structure of a canonical PARG from T. thermophila The full-length TTPARG is highly similar to the minimal catalytic region of human PARG, but it lacks the obvious RS/MTS motif ( Fig. 1a ; Supplementary Fig. S1 ). Nonetheless, the TTPARG binds ADP-ribose ( Supplementary Fig. S2 ) and displays high PAR glycohydrolase activity. This activity is dependent on the conserved glutamate residues as observed for other PARGs ( Fig. 1b ). 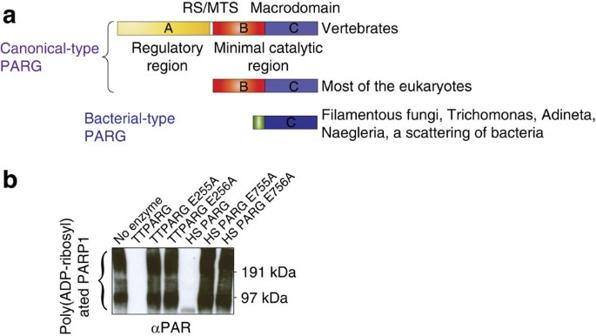Figure 1: Phylogenetic distribution and the activity of PARG enzymes. (a) The domain structure of canonical and bacterial type PARGs. (b) Poly(ADP-ribose) hydrolytic activities ofTetrahymena thermophilaand human PARGs. The activity is dependent on the integrity of catalytic glutamate residues. The structure was solved using a Se-Met MAD-based approach and refined against 1.95 Å data ( Table 1 ; Supplementary Fig. S3 ). The TTPARG structure ( Fig. 2 ) consists of a macrodomain sandwiched between a large N-terminal accessory domain and a smaller carboxy-terminal extension. The macrodomain itself is most similar in structure to the recently determined bacterial PARG (bactPARG) structure ( Fig. 2b ; PDB code 3SIG Z score 15.4), with which it shares the PARG-specific loop. In both bacterial and TTPARG, the conformation of the glycine-rich PARG catalytic loop seems to be stabilized by contacts with residues derived from an N-terminal extension to the macrodomain. In bactPARG, this extension consists of a few α-helices ( Fig. 2b ). In contrast, the N-terminal accessory domain of the TTPARG accounts for approximately half of the enzyme structure and is predominantly α-helical in nature, with the exception of a few β-strands that form an extension to the macrodomain central β-sheet. This accessory domain is not related to any previously determined structures and seems unique to canonical PARGs. Given the sequence similarity between human and Tetrahymena PARGs (32% identity for residues 91–431), a plausible model (r.m.s.d. 0.51 Å) can be created accounting for the majority of the human PARG catalytic domain (residues 604–937) ( Fig. 2c ). We attempted to produce truncations in the N-terminal domain of TTPARG, which were chosen based on our structure (Δ1-67 and Δ1-115), but both truncations dramatically affected expression and stability of the proteins in Escherichia coli . Similar behaviour was observed for homologous truncations of human PARG, demonstrating the importance of the N-terminal domain for canonical PARGs. Despite this, we obtained some soluble protein for the human PARG truncation Δ1-619 (corresponding to TTPARG Δ1-115), and this protein exhibited significant PARG activity in vitro ( Supplementary Fig. S4 ), demonstrating that the RS/MTS motif [14] and a large part of the N-terminal domain are not absolutely essential for the enzymatic activity of canonical PARGs. Figure 1: Phylogenetic distribution and the activity of PARG enzymes. ( a ) The domain structure of canonical and bacterial type PARGs. ( b ) Poly(ADP-ribose) hydrolytic activities of Tetrahymena thermophila and human PARGs. The activity is dependent on the integrity of catalytic glutamate residues. Full size image Table 1 Data collection and refinement statistics. 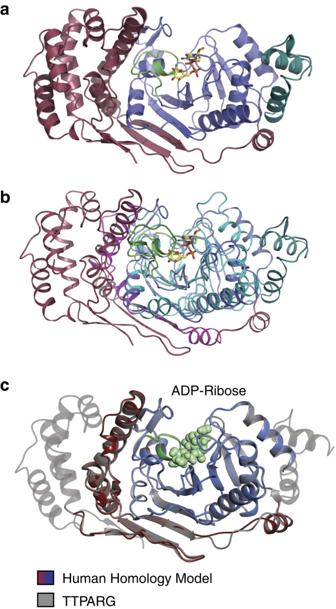Figure 2: Structure of canonical PARG enzyme fromTetrahymena thermophila. (a) The TTPARG-ADP-ribose complex structure. The TTPARG macrodomain is coloured in blue (residues 218–414), the catalytic PARG loop in green (residues 244–256), the N-terminal accessory domain in red (residues 1–217), and the C-terminal extension in teal (residues 415–458). (b) A TTPARG/bactPARG structure overlay. TTPARG is coloured as in (a). The bactPARG structure is shown using cyan for the macrodomain, magenta for the N-terminal extension, and a dark green colour for the catalytic PARG loop. (c) Homology model for the human PARG catalytic domain, using residues 91–431 of TTPARG as a template, for clarity, regions not included in the model (due to lack of significant homology in those regions) are transparent. Full size table Figure 2: Structure of canonical PARG enzyme from Tetrahymena thermophila . ( a ) The TTPARG-ADP-ribose complex structure. The TTPARG macrodomain is coloured in blue (residues 218–414), the catalytic PARG loop in green (residues 244–256), the N-terminal accessory domain in red (residues 1–217), and the C-terminal extension in teal (residues 415–458). ( b ) A TTPARG/bactPARG structure overlay. TTPARG is coloured as in ( a ). The bactPARG structure is shown using cyan for the macrodomain, magenta for the N-terminal extension, and a dark green colour for the catalytic PARG loop. ( c ) Homology model for the human PARG catalytic domain, using residues 91–431 of TTPARG as a template, for clarity, regions not included in the model (due to lack of significant homology in those regions) are transparent. Full size image The canonical PARG catalytic mechanism The TTPARG active site is clearly identified by the presence of the ADP-ribose ligand ( Fig. 3a ). The ADP-moiety is bound by the macrodomain with the ribose group located in close proximity to the key catalytic residues provided by the PARG-specific catalytic loop. Our homology model reveals that near-identical contacts occur in the human PARG ( Fig. 3b ). The majority of the hydrogen bonds established with the ligand phosphates occur through main chain atoms. The adenosine base is stacked with Phe398 and forms direct hydrogen bonds with Ile227 and Glu228. Whereas the C2-hydroxyl group of the adenosine ribose is devoid of any protein-ligand interactions, a water-mediated network of interactions can be observed for the C3-hydroxyl group. This network includes the Y296 side chain, homologous to the hPARG Y795 previously implicated in the binding of an ADP-ribose analogue inhibitor of PARG [15] . Mutation of this residue leads to reduced PARG activity in vitro for both TTPARG and hPARG ( Fig. 3c ; Supplementary Fig. S5 ). Each of the ribose hydroxyl groups is directly hydrogen-bonded by a PARG residue, with C1, C2 and C3 hydroxyl groups bound by Glu256, Glu255 and Asn240, respectively. While mutation of the conserved Glu residues abolishes enzyme activity, Asn240Ala (Asn740Ala in hPARG) mutants retain a low level of in vitro activity ( Fig. 3c ). Glu255 is in direct hydrogen-bonding contact with Asp237, which has been previously implicated in canonical PARG activity [5] . The ribose' moiety is also in direct van der Waals contact with Phe371. This interaction is important for the activity, as Phe371Ala (Phe875Ala in hPARG) severely affects the ability of the enzyme to hydrolyse PAR ( Fig. 3c ). 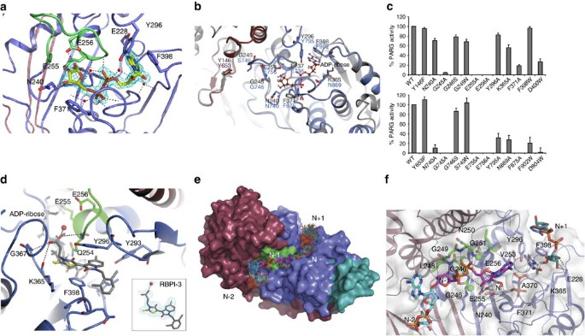Figure 3: Reaction mechanism of canonical PARGs. (a) Bound ADP-ribose is shown with electron density in cyan. For clarity, interactions with backbone are only indicated by dotted lines, with no representation of the backbone atoms. (b) Detailed view of the active site regions of the human PARG homology model (in grey), overlayed with the corresponding TTPARG structure. (c) Relative poly(ADP-ribose) hydrolytic activities ofTetrahymena thermophila(upper panel) and human (lower panel) PARG mutants. Error bars represent s.d. (n=3). (d) Structure of the TTPARG-RBPI-3 complex. RBPI-3 is shown in atom-coloured sticks, with an ADP ribose overlayed in black. The omit 2Fo-Fcelectron density corresponding to RBPI-3 is shown in the insert as a blue mesh contoured at 1.5σ. (e) A PARG-PAR4model surface representation of TTPARG with 40 different PAR4conformations derived from MD simulations. The PAR4is shown in atom-colored sticks with ADP-ribose N in grey carbons, N−1 magenta carbons, N−2 teal carbons and N+1 in green carbons. (f) Detailed view of the PAR-binding site of a representative PARG-PAR4model. The PAR4is coloured as in (a), with key contacts between PARG-PAR4displayed by black dotted lines. Cα atoms of Gly residues important in PAR4binding are shown in spheres. Figure 3: Reaction mechanism of canonical PARGs. ( a ) Bound ADP-ribose is shown with electron density in cyan. For clarity, interactions with backbone are only indicated by dotted lines, with no representation of the backbone atoms. ( b ) Detailed view of the active site regions of the human PARG homology model (in grey), overlayed with the corresponding TTPARG structure. ( c ) Relative poly(ADP-ribose) hydrolytic activities of Tetrahymena thermophila (upper panel) and human (lower panel) PARG mutants. Error bars represent s.d. ( n =3). ( d ) Structure of the TTPARG-RBPI-3 complex. RBPI-3 is shown in atom-coloured sticks, with an ADP ribose overlayed in black. The omit 2 Fo - Fc electron density corresponding to RBPI-3 is shown in the insert as a blue mesh contoured at 1.5σ. ( e ) A PARG-PAR 4 model surface representation of TTPARG with 40 different PAR 4 conformations derived from MD simulations. The PAR 4 is shown in atom-colored sticks with ADP-ribose N in grey carbons, N−1 magenta carbons, N−2 teal carbons and N+1 in green carbons. ( f ) Detailed view of the PAR-binding site of a representative PARG-PAR 4 model. The PAR 4 is coloured as in ( a ), with key contacts between PARG-PAR 4 displayed by black dotted lines. Cα atoms of Gly residues important in PAR 4 binding are shown in spheres. Full size image A comparison with the previously determined bactPARG-ADP-ribose complex structure reveals significant similarity in enzyme-ligand interactions between both complexes ( Supplementary Fig. S6 ). In both enzymes, the Gly-rich PARG catalytic loop conformation is stabilized through interactions with residues from an N-terminal extension to the macrodomain. The catalytic Glu residues bind the ribose C1 and C2 hydroxyl groups, with Glu256 (Glu756 in hPARG) presumably acting as the hydrogen donor to the leaving group. The Asp237–Glu255 pair could form a proton relay network to Glu256, mediated in part by the ADP-ribose hydroxyl groups. In bactPARG, Asn95 replaces the TTPARG Asp237, which suggests that the mechanism for PAR hydrolysis is subtly different between both enzymes, or that TTPARG Glu255 and/or bactPARG Glu114 are not directly involved in acid-base catalysis. Regardless, in both enzymes, the transient oxocarbenium intermediate seems to be stabilized by close contact with the adenosine diphosphate group, an interaction enforced by the presence of Phe371 (Phe227 in bactPARG). In both structures, a water molecule is positioned in close contact to the C1 carbon, with nucleophilic attack on C1 facilitated by Glu256 (Glu115 in bactPARG) acting as a base. Structure of a mammalian PARG inhibitor:TTPARG complex Inhibition of mammalian PARG enzymes was recently shown for several related rhodanine-containing compounds [16] . Not unexpectedly, we were able to show that TTPARG is also inhibited by this class of inhibitors ( Supplementary Fig. S7 ). The structure of the TTPARG-inhibitor complex obtained by co-crystallization reveals that the inhibitor RBPI-3 binds predominantly via a π–π stacking interaction with Tyr296 (implicated in binding of distinct ADP-ribose analogues [15] ) and the conserved Phe398 ( Fig. 3d ). To accommodate the binding of RBPI-3, Phe398 moves into the adenosine binding pocket. The RBPI-3 carboxyl moiety occupies a region corresponding to the ADP-ribose alpha-phosphate group and H-bonds to main chain atoms of Lys365 and Gln254. The RBPI-3 di-chlorobenzyl moiety extends into the solvent and is disordered. Poly(ADP-ribose) recognition by canonical PARGs To further explore canonical PARG-PAR interactions, we modelled an oligo(ADP-ribose) 4 molecule in the TTPARG structure ( Fig. 3e,f ). The position and conformation of the n −1, n −2 and n +1 ADP-ribose units ( n being the ADP-ribose unit observed in the crystal structure) can be derived from linking these through an α(O1 ribose' -O2 ribose ) O -glycosidic linkage and through the constraints imposed on the available space by the TTPARG structure. The model predicts that the n −1 ribose unit is in van der Waals contact with both Gly246 and Gly251, whereas the n −1 adenosine base is sandwiched against Val253 and Ala370. The n –1 diphosphate group is located in close proximity to the conserved Gly246, with the α-phosphate, making polar contacts with the amide nitrogens of Asn250 and Gly251. Molecular dynamics simulations suggest that the PAR ligand shows significant mobility from the n −1 β-phosphate, with increasing conformational flexibility for the n −1 ribose and n −2 ADP-ribose unit ( Fig. 3e ). Mutation of Gly246 to Ser (G746S in hPARG) leads to a significant reduction in in vitro activity, while the effect of mutating the preceding Gly245 to Ala (G745A in hPARG) nearly completely abolishes activity ( Fig. 3c ). The Cα of the latter residue is van der Waals contact with the n -ribose O2 group. This suggests that binding, and/or orientation, of the n −1 ADP-ribose is less critical to activity when compared with binding of the n ADP-ribose. The n −2 ADP-ribose is only contacted by residues from the N-terminal accessory domain, where sequence conservation is limited compared with those regions contacting the n −1 and n units, and it displays significant conformational mobility ( Fig. 3e ). The adenosine C2-hydroxyl group is solvent exposed in the TTPARG structure, in contrast to bactPARG, and modelling of an additional n +1 ADP-ribose reveals that TTPARG can bind PAR at intermediate positions, and could thus display endo-glycohydrolase activity as suggested for canonical PARGs [17] . However, the endo-glycohydrolase activity has been very difficult to confirm, as it was suggested to be coupled with exo-glycohydrolase activity [18] . Thus far, we have not been able to experimentally demonstrate the endo-glycohydrolase activity for any of our PARG enzyme preparations and we consistently observed ADP-ribose as the only detectable product ( Supplementary Fig. S8 ) [10] . Nonetheless, we tested some mutants at the n +1 ADP-ribose binding site that, according to our PAR-PARG model, could specifically affect the endo-glycohydrolase function. For example, the ribose' of the n +1 ADP-ribose is positioned in close contact with Lys365, which can hydrogen-bond to both C2 and C3 hydroxyl groups. Interestingly, the mutation of Lys365 to Ala (Asn869Ala in hPARG) leads to diminished in vitro activity while retaining ADP-ribose-binding properties, as verified by thermal shift assays ( Fig. 3c; Supplementary Fig. S9 ). We also analysed the effect of mutating Phe398 and Asp400 to tryptophan that based on our predictions could affect the TTPARG endo-glycohydrolase function by blocking the binding to n +1 ADP-ribose. We observed a substantially reduced overall PARG activity for the Asp400Trp TTPARG mutant only ( Fig. 3c ; Supplementary Fig. S9 ). Mutating the homologous residues in human PARG in both cases severely affected the activity of the protein. Collectively, our model suggests that canonical PARG-PAR specific contacts are more extensive than for bactPARG, but are still limited to the n and, to a lesser extent, n −1 and n +1 ADP-ribose units. In summary, we reveal the first structure of a canonical PARG. Our data suggests that canonical PARG is similar in mechanism to bacterial-type PARGs, but displays some key differences, including additional PAR-PARG interactions (that is, Asn240, Tyr296 and Lys365) and the ability to bind PAR at intermediate positions. Targeting poly(ADP-ribosyl)ation in the therapy of human disease has attracted considerable attention over the past few years after it was demonstrated that permeable PARP inhibitors can be highly effective against hereditary breast and ovarian cancers [19] . Given the impact and the prevalence of these diseases, there has been a rapidly growing interest in PARG as an alternative target in human therapy. We believe that the novel PARG-inhibitor structure presented here could provide the groundwork for future studies that might lead to the development of small, cell-permeable PARG inhibitors. Plasmids and proteins The T. thermophila PARG2 (TTHERM_00294690) was synthesized, according to the database sequence (GenScript USA). The human PARG gene (Q86W56) was cloned from HeLa complementary DNA. T. thermophila PARG proteins were expressed from the pET28a vector (Novagen). Human PARG with an N-terminal truncation (Δ1-455) served as a reference for the wild-type PARG activity and the mutant PARG constructs were expressed from the pColdTF vector (Takara). All proteins bear an N-terminal his tag. Human proteins bear the additional Trigger Factor chaperone tag that increases solubility. Mutations were introduced using the QuickChange II site-directed mutagenesis kit (Stratagene). Proteins were expressed in E. coli Rosetta2(DE3) cells (Novagen). Recombinant proteins were purified on Ni-NTA beads, according to standard procedure. For crystallization studies, the T. thermophila PARG2 was purified by FPLC on a HisTrap HP column followed by gel filtration, using HiLoad 16/60 Superdex 200 column (GE Healthcare). Rhodanine-containing PARG inhibitor RBPI-3 was synthetized, as described [16] . PARG activity assays For western-blot analysis of PARG activity, poly(ADP-ribose) was synthesized by the automodification of PARP1 in a reaction mixture containing 2 units of PARP1 (Trevigen), 200 μM NAD (Trevigen), activated DNA (Trevigen), 50 mM Tris pH 7.5. and 50 mM NaCl at room temperature. Reactions were stopped after 30 min by the addition of the PARP inhibitor KU-0058948. In reactions, either 1 μM of both human and T. thermophila PARGs, or for mutational analysis, 400 nM human and 30 nM T. thermophila PARGs were added to the reaction and incubated for another 30 min. The reactions were run on 4–12% SDS–PAGE gels and blotted onto a nitrocellulose membrane. PAR hydrolysis was detected by rabbit polyclonal anti-PAR antibodies (Trevigen; 1:1,000 dilution). Western blots were analysed densitometrically by GeneTools (SynGene). PARG inhibition assay Inhibition of TTPARG by RBPI-3 was determined, as previously reported [16] , with the following modifications. Purified TTPARG was employed at a final concentration of 50 nM and reactions were incubated at 37 °C for 60 min before stopping by the addition of 1.0 μl 1% SDS. Thermal shift assay In each 50 μl reaction, 15 μl of 300× Sypro Orange (Sigma), 2 μl of water and 33 μl of protein (4 mg ml −1 ) in 25 mm Tris pH 7.5, 50 mM NaCl, 10% glycerol and 1 mM DTT were added to the wells of a 96-well thin-wall PCR plate (Bio-Rad). For thermal shift assays in the presence of ADP-ribose, 2 μl of 25 mM ADP-ribose was added instead of water. Samples were placed in a CFX96 Real-Time PCR thermal cycler (Bio-Rad) and slowly heated from 15 to 95 °C with sample fluorescence recorded every 0.2 °C. Fluorescence was monitored at 575 nm (emission), using 490 nm for excitation. Protein expression and purification Selenomethionine TTPARG was produced in the same Rosetta (DE3) cells as native TTPARG, but in the conditions where the methionine biosynthesis pathway is inhibited [20] . Briefly, 1 l of unlabelled TBGG ('Terrific Broth' supplemented with 1.0% glucose and 4% glycerol) was inoculated with 5 ml of an overnight culture grown in lysogeny broth (LB). The culture was grown to mid-log phase, pelleted and washed. The pellet was resuspended in warm minimal media and evenly distributed between 6 l of Se-Met supplemented media—Se-Met media contains abundant amounts of all amino acids known to inhibit methionine biosynthesis but no methionine (1.8 g of all amino acids). Finally, 50 mg of Selenomethionine was added and the cultures allowed to recover for 90 min before being induced with 1 mm isopropyl-β- D -thiogalactoside overnight at 30 °C. The native and selenomethionine-labelled proteins were purified to homogeneity by HisTrap HP Ni 2+ -affinity chromatography followed by size exclusion chromatography on a HiLoad 16/60 Superdex 200 column. Samples were concentrated to ~15 mg ml −1 and 1:1 molar ratio of TTPARG to ADP-ribose was added before crystallization experiments. Structure determination and refinement Selenomethionine incorporated TTPARG crystals were obtained by sitting drop vapour diffusion in drops containing equal volumes of ADP-ribose complexed protein and a solution containing 0.15 M potassium thiocyanate, 0.1 M Tris pH 8.5 and 15% PEG 6 K. Data was obtained on beamline IO4 at the Diamond light source and reduced and scaled with the X-ray Detector Software suite. The crystal structure of TTPARG was determined by Single-wavelength anomalous diffraction and was phased with the program Solve [21] . The resulting map allowed a single low-resolution copy of TTPARG to be built with Bucanneer [22] . An additional high-resolution data set was collected, on a second crystal grown in conditions containing 0.2 M potassium bromide, 0.1 M Tris pH7.5 and 15% PEG 4 K. The low-resolution model from Buccaneer was then used as a start model for molecular replacement and applied to the high-resolution data. The resulting MR solution contained two TTPARG molecules in the asymmetric unit (AU). The missing residues and loops were completed by iterative cycles of automated model building (ARP/wARP) and manual model building and real-space refinement, using the program COOT and crystallographic refinement using phenix.refine. Structure validation was preformed with Molprobity. Co-crystallization with the RBPI-3 inhibitor was carried out by replacing ADP-ribose with RBPI-3. The processing and final refinement statistics are presented in Table 1 . The thermodynamic ligand-binding properties of TTPARG and ADP-ribose was measured using a VP-ITC microcalorimeter. Protein and ligand concentrations were 20 μM and 200 μM, respectively in 50 mM Tris (pH 7.5), 100 mM NaCl. Titration curves were fitted using a nonlinear least-squares method in Microcal Origin software. A model that was indicative of a single-binding site was found to give the best fit and this model was used to obtain the thermodynamic parameters. Computational simulations NAMD software [23] was used to perform all molecular dynamics (MD) simulations of the ADP-α-ribose tetramer in complex with PARG [10] . PAR tetramer was created by addition of three additional ADP-a-ribose monomers to the ADP-a-ribose bound to PARG. Topology, and parameters files for this ligand were obtained using Antechamber program [24] and AM1-BCC charges [25] . The PARG-tetramer complex model was immersed in a periodic water box (TIP3) and neutralized by adding Na + ions. This complex was equilibrated with several cycles of minimizations (steepest descent, 10,000 steps) and MD simulations (50 K, 20 ps) with the protein atoms kept fixed. Then MD simulations were performed (200 K, 2 ns), with the protein backbone restrained on the X-ray structure conformation. During these MD simulations, several snapshots were periodically extracted and energy-minimized (no restraints) to show the binding interactions of PAR tetramer with PARG active site. Analyses by ultrahigh-performance liquid chromatography The poly(ADP-ribosyl)ated PARP1 was treated with PARG, and the mixture filtered using centricons (30 kDa cutoff). The analysis of the filtrate was performed using a modified procedure by Coulier et al . [26] , which employed ion-pair chromatography for the separation of nucleotides and negative electrospray ionization for the mass spectrometric detection. All analyses were performed using a Waters Acquity UPLC system (Waters Corp., Milford, MA, USA) coupled to a QTOF Premier mass spectrometer (Waters Micromass, Manchester, UK). The chromatographic separations employed a column (100 mm×2.1 mm) filled with a 1.7-μm BEH C18 stationary phase (Waters Corp., Milford, MA, USA). Binary gradients at a flow rate of 0.4 ml min −1 were applied for the elution. The eluent A was water containing 5 mmol l −1 of pentylamine with the pH value adjusted to 6.5, using acetic acid. The eluent B was acetonitrile. A fast elution gradient was applied, starting with 2% B and then the percentage of B linearly increased to 25% in 5 min, followed by an isocratic hold until 9 min. The mass spectrometry was performed using an orthogonal Z-spray-electrospray interface. Drying gas and nebulizing gas was nitrogen. The desolvation gas flow was set to 700 l h −1 at a temperature of 280 °C. The cone gas flow was adjusted to 25 l h −1 , and the source temperature to 120 °C. The capillary and cone voltages were 3,500 V and 30 V, respectively. The instrument was operated in V mode with TOFMS data being collected between m/z 100–2,000, applying collision energy of 4 eV. Leucine enkephalin was applied as a lock mass in negative ionization mode (m/z 554.2615). The chromatograms, recorded in the total ion current mode, were systematically examined by manually generating mass spectra of each visible individual peak using background-subtraction option. Specific target components, expected to occur in the reaction mixture, in particular ADP-ribose, oligomers of poly ADP-ribose with up to 5 ADP-ribose units and NAD + , were searched for using extracted ion chromatograms. The target analyses were based on the accurate mass feature of the instrument, applying a mass window of 50 mDa. Information on the electrospray ionization mass spectra for oligomeric ADP-ribose species is only scarcely available in the literature [27] . Therefore, the recorded total ion current chromatograms were systematically examined using specific masses of possible mono- and multiply charged ions of individual oligomers. Accession codes: Atomic coordinates and structure factors have been deposited in the Protein Data Bank under accession codes 4EPP and 4EPQ How to cite this article: Dunstan, M. S. et al . Structure and mechanism of a canonical poly(ADP-ribose) glycohydrolase. Nat. Commun. 3:878 doi: 10.1038/ncomms1889 (2012).